Stretchable chiral pockets for palladium-catalyzed highly chemo- and enantioselective allenylation Pyrazolones are a vital class of heterocycles possessing various biological properties and much attention is paid to the diversified synthesis of enantiopure pyrazolone derivatives. We describe here the development of diphenylphosphinoalkanoic acid based chiral bisphosphine ligands, which are successfully applied to the palladium-catalyzed asymmetric allenylation of racemic pyrazol-5-ones. The reaction affords C-allenylation products, optically active pyrazol-5-ones bearing an allene unit, in high chemo- and enantioselectivity, with DACH-ZYC-Phos-C1 as the best ligand. The synthetic potential of the C-allenylation products is demonstrated. Furthermore, the enantioselectivity observed with DACH-ZYC-Phos-C1 is rationalized by density functional theory studies. Pyrazolones are a vital class of heterocycles possessing various biological properties [1] . Of particular interest are the pyrazolone derivatives with a chiral center (Fig. 1a ): compound A and its derivatives were proven to be orally active growth hormone secretagogues [2] , [3] ; compound B was used as a modulator of TRPM8; [4] compound C shows remarkable anti-tumor activity related to lung, colon, and breast cancer cell [5] , [6] . Thus, much attention has been paid to the diversified synthesis of bioactive enantiopure pyrazolone derivatives [7] , [8] , [9] , [10] , [11] , [12] , [13] , [14] , [15] , [16] , [17] , [18] , [19] , [20] , [21] , [22] , [23] , [24] , [25] , [26] , [27] . Along this line, enatioselective allylation of pyrazolones has been established [9] , [10] , [11] , [12] . For allene derivatives, enatioseletive spirocyclizations of pyrazolones with 2,3-allenyl acetates have been developed by applying chiral phosphine or transmetal/chiral ligand catalysis (Fig. 1b ) [13] , [14] . So far, there is no report on enantioselective 2,3-allenylation of pyrazolones, which is very attractive owing to the unique biological [28] , [29] , [30] and chemical properties [31] , [32] , [33] , [34] , [35] , [36] , [37] of the allene unit and pyrazolone moiety. Fig. 1: Background and stretchable ligands for asymmetric allenylation of pyrazolones. a Selected examples of biologically active pyrazolones with a chiral center. b Asymmetric spirocyclization of pyrazolones with 2,3-allenyl acetates. c Stretchable chiral pocket for asymmetric allenylation. EWG electron-withdrawing group, TMS trimethylsilyl, LG leaving group. Full size image In this work, inspired by conformationally flexible alkyl chain in the Feng’s ligands, we develop the enantioselective allenylation of pyrazolones by fine tuning of the Trost ligands, which leads to the development of a class of stretchable chiral pocket (Fig. 1c ). Initially, we studied the enantioselective allenylation of pyrazol-5-one 2a with benzyl 2-butylbuta-2,3-dienyl carbonate 1a with some typical and commercially available chiral ligands at 30 °C in CHCl 3 (Fig. 2 ). With L1 and L8 as the ligand, there was a serious competing reaction forming N -allenylation product 4aa . Further screening led to the observation that L2 – L7 were sluggish for this allenylation. In the reaction with Trost ligand L9 , no product was observed, while Trost ligand L10 afforded the C-allenylation product ( S )- 3aa in 73% yield and 50% ee; interestingly, Trost ligand L11 could give ( S )- 3aa in 84% yield and 75% ee. With L11 as the ligand, subsequent investigation on the solvent effect showed that toluene was the best one, affording 85% yield ( S )- 3aa with 84% ee (Fig. 2 , entries 1–5). After optimizing the temperature and concentration (Fig. 2 , entries 6–11), the reaction at 0.02 M could give ( S )- 3aa in 92% yield and 85% ee, together with a trace amount of 4aa at 60 °C (Fig. 2 , entry 11). Fig. 2: The selected data of optimization with some commercially available chiral ligands. a Reaction conditions: 1a (0.2 mmol), 2a (1.2 equiv), Pd 2 (dba) 3 •CHCl 3 (2.5 mol%), and L1 - 4 (12 mol%) or L5 - 11 (6 mol%) unless otherwise noted. b The yields of ( S )- 3aa and 4aa as well as the recovery of 1a were determined by the 1 H NMR analysis of the crude product using mesitylene as the internal standard and the ee of isolated ( S )- 3aa was determined by chiral HPLC. c The reaction time was 4 h. d L11 (5 mol%) was used and the reaction time was 3 h. Cbz benzyloxycarbonyl, THF tetrahydrofuran, DMF N , N -dimethylformamide, n.d. not determined. Full size image Obviously, a higher enantioselectivity was desired and the success of conformationally flexible alkyl chain in the Feng’s ligands [38] , [39] , [40] , [41] has caught our attention (Fig. 3a ). It was reasoned that the rigid aryl linker in the Trost ligands may be replaced with a flexible alkyl linker for a class of stretchable chiral pockets seeking higher enantioselectivity. Thus, the ZYC-Phos ligands were designed and readily synthesized by amidation of diphenylphosphino alkanoic acids, which were prepared by nucleophilic substitution of ethyl chloroalkanoate or chloroacetic acid (Fig. 3b ) for further optimization [42] , [43] , [44] , [45] . Fig. 3: Concept and synthesis of the ZYC-Phos ligands. a The concept of ZYC-Phos ligands from the Feng’s ligands and the Trost ligands. b The synthesis of ZYC-Phos ligands. EDCI 1-ethyl-(3-dimethylaminipropyl)carbodiimide hydrochloride, NHS N -hydroxysuccinimde, DMSO dimethyl sulfoxide, DCM dichloromethane, DACH (1 R ,2 R )-1,2-diaminocyclohexane, DADPE (1 R ,2 R )-1,2-diphenyl-1,2-diaminoethane, DMAP 4-dimethylaminopyridine. Full size image With the ligands in hand, we conducted the allenylation with DACH-ZYC-Phos-C2 . 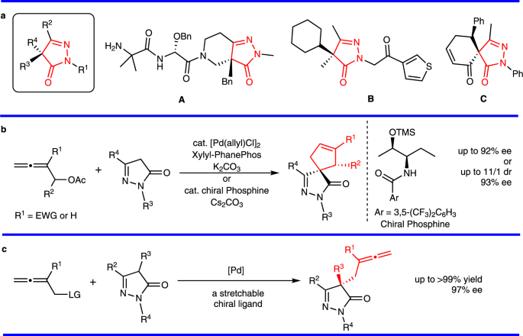Fig. 1: Background and stretchable ligands for asymmetric allenylation of pyrazolones. aSelected examples of biologically active pyrazolones with a chiral center.bAsymmetric spirocyclization of pyrazolones with 2,3-allenyl acetates.cStretchable chiral pocket for asymmetric allenylation. EWG electron-withdrawing group, TMS trimethylsilyl, LG leaving group. The reaction afforded ( S )- 3aa in 85% ee, albeit with a low conversion (14% yield with 67% recovery of 1a ) (Table 1 , entry 1). Further optiminization was performed: the reactions at 60 °C and 80 °C afforded ( S )- 3aa in 75 and 80% yields, respectively, with a similar ee together with 4% of the N -allenylation product 4aa (Table 1 , entries 2 and 3). Next, we investigated the effect of concentration (Table 1 , entries 4–6) and observed that the ee of ( S )- 3aa was improved to 88% when the concentration of the reaction was 0.02 M. The ee value of ( S )- 3aa was similar with 5.0 mol% of the ligand (Table 1 , entry 7). DADPE-ZYC-Phos-C2 , DACH-ZYC-Phos-C3 , and DACH-ZYC-Phos-C1 (Table 1 , entries 8–10) were then screened and DACH-ZYC-Phos-C1 was found to afford ( S )- 3aa in 79% yield and 90% ee as the chiral ligand with 2% of N -allenylation product 4aa . Solvent screening (Table 1 , entries 11–13) led to the conclusion that toluene was the best choice, exclusively affording ( S )- 3aa in 100% yield and 95% ee. Using toluene as solvent, DACH-ZYC-Phos-C2 and C3 were re-tested (Table 1 , entries 14 and 15). Thus, the optimal conditions were redefined as follows: allene 1 , pyrazolone 2 (1.2 equiv), Pd 2 (dba) 3 •CHCl 3 (2.5 mol%), and DACH-ZYC-Phos-C1 (5.0 mol%) in toluene (0.02 M) at 60 °C (Table 1 , entry 11). Table 1 The effect of temperature, concentration, ligands, and solvents on the asymmetric allenylation of pyrazolone 2a with allene 1a a . Full size table The scope of benzyl buta-2,3-dienyl carbonates 1 was then examined with pyrazol-5-one 2a . 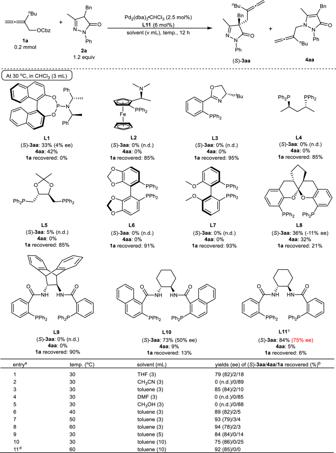Fig. 2: The selected data of optimization with some commercially available chiral ligands. aReaction conditions:1a(0.2 mmol),2a(1.2 equiv), Pd2(dba)3•CHCl3(2.5 mol%), andL1-4(12 mol%) orL5-11(6 mol%) unless otherwise noted.bThe yields of (S)-3aaand4aaas well as the recovery of1awere determined by the1H NMR analysis of the crude product using mesitylene as the internal standard and the ee of isolated (S)-3aawas determined by chiral HPLC.cThe reaction time was 4 h.dL11(5 mol%) was used and the reaction time was 3 h. Cbz benzyloxycarbonyl, THF tetrahydrofuran, DMFN,N-dimethylformamide, n.d. not determined. For R 1 , n -butyl, methyl, n -octyl, TMS, and phenyl all worked well with an excellent yield and ee (Table 2 , entries 1–5). However, when R 1 is H, the ee value of ( R )- 3fa dropped to 78% with 86% yield, indicating a serious steric effect (Table 2 , entry 6). The scope of pyrazol-5-ones 2 was then examined with benzyl 2-( n -butyl)buta-2,3-dienyl carbonate 1a . 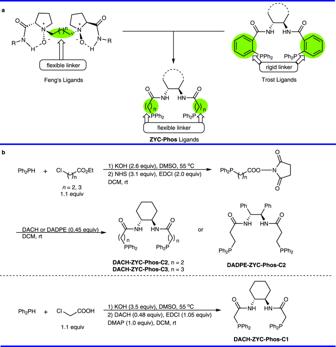Fig. 3: Concept and synthesis of the ZYC-Phos ligands. aThe concept ofZYC-Phosligands from the Feng’s ligands and the Trost ligands.bThe synthesis ofZYC-Phosligands. EDCI 1-ethyl-(3-dimethylaminipropyl)carbodiimide hydrochloride, NHSN-hydroxysuccinimde, DMSO dimethyl sulfoxide, DCM dichloromethane, DACH (1R,2R)-1,2-diaminocyclohexane, DADPE (1R,2R)-1,2-diphenyl-1,2-diaminoethane, DMAP 4-dimethylaminopyridine. The reaction of 4-( ortho- , meta - or para -methylbenzyl)pyrazol-5-ones 2b – 2d with 1a afforded ( R )- 3ab ~( S )- 3ad in similar yields and enantioselectivity (Table 2 , entries 7–9), suggesting that the location of the substituent on the aryl group in the 4-benzyl unit has very limited effect for enantioselectivity. Some synthetic versatile functionalities, such as Cl, Br, F, CN, CF 3 , MeO, and NO 2 , survived well in the reaction of 1a and pyrazol-5-ones 2 , affording ( S )- 3ae ~( S )- 3ak in 86–97% yields and 94–98% ee (Table 2 , entries 10–16). The absolute configuration was determined by the X-ray single crystal diffraction analysis of ( S )- 3ak (Fig. 4a ). Furthermore, 4-ethyl, 4-allyl, and 4-(α-naphthylmethyl)pyrazol-5-ones 2l – 2n were exercisable with 87–96% yields and 93–97% ee (Table 2 , entries 17, 18, 20). As expected, enantiomer ( R )- 3am was obtained in 95% yield and 94% ee by using ent - DACH-ZYC-Phos-C1 as the ligand (Table 2 , entry 19). It should be noted that the difference between the ee values of ( R )- 3ao and ( R )- 3ap suggested that coordination of the hydroxyl oxygen may affect the enantioselectivity (Table 2 , entries 21 and 22). Furthermore, for R 3 being phenyl, the ee value of ( R )- 3at was only 36% with 62% yield (Table 2 , entry 23). 3-Ethyl, 3-isopropyl, and 3-phenyl pyrazol-5-ones 2q – 2s also worked smoothly to offer the products in 91–>99% yields and 95–97% ee (Table 2 , entries 24–26). The reaction of N -cyclohexyl pyrazol-5-one 2 u and 1b afforded ( S )- 3bu in 84% yield with 95% ee while the reaction of N -benzyl pyrazol-5-one 2 v and 1b afforded ( S )- 3bv in 82% yield with 90% ee (Table 2 , entries 27 and 28). Table 2 The scope of allenes and pyrazol-5-ones a . Full size table Fig. 4: ORTEP representation and sythetic applications. a ORTEP representation of ( S )- 3ak . b The gram-scale reaction and applications: reaction conditions: (i) Pd 2 (dba) 3 •CHCl 3 (2.5 mol%), DACH-ZYC-Phos-C1 (5.0 mol%), toluene, 60 °C, 13 h; (ii) [Rh(CO) 2 Cl] 2 (5.0 mol%), AgSbF 6 (12.5 mol%), CO balloon, toluene, 50 °C, 13 h; (iii) ortho-(propen-2-yl)phenol (3.0 equiv), Pd(OAc) 2 (7.5 mol%), 2,2’-bipy (7.5 mol%), Cu(OAc) 2 •H 2 O (0.5 equiv), toluene, 110 °C, 18 h; (iv) TiCl 4 (1.5 equiv), dichloromethane, −78 °C, 2.5 h, rt, 5.5 h. TMS trimethylsilyl, Cbz benzyloxycarbonyl, y. isolated yield. Full size image The reaction of 1a and 2 m could be conducted on gram scale facilely, affording 1.20 g of ( S )- 3am in a similar yield and enantioselectivity (Fig. 4b–i ). Subsequently, an allenic Pauson–Khand annulation of ( S )- 3am was established in 55% yield and 99% ee to afford tricyclic product (3a S ,5 S )- 5am containing a bicyclic motif with anti-tumor activity [46] (see compound C in Fig. 1a ). The annulation reaction of ( S )- 3da with o -(propen-2-yl)phenol could easily construct a seven-membered heterocycle in product ( S , Z )- 6da (72% yield, 95% ee and > 20/1 Z / E ) [47] . The allene unit in ( S )- 3da also could be transformed into a 2-propynyl side chain in ( S )- 7da upon treatment with TiCl 4 . A possible mechanism for the allenylation of pyrazolone is shown in Fig. 5a [48] , [49] , [50] . To better understand the superior enatioselectivity and the advantage of DACH-ZYC-Phos-C1 in the allenylation of pyrazolone, we have conducted X-ray single crystal diffraction studies: firstly, Pd(II)- DACH-ZYC-Phos-C1 complex ( III ) was prepared by the reaction of PdCl 2 and DACH-ZYC-Phos-C1 with excess amount of bases in toluene (Fig. 5b ). Pd(II)-DACH-Phenyl Trost ligand complex ( IV ) was obtained from the reaction of Pd(OAc) 2 with DACH-Phenyl Trost ligand with excess amount of bases in THF [51] . Both complexes were then recrystalized from CHCl 3 / n -hexane to afford single crystals suitable for the X-ray diffraction study. It was obvious that the angle (P1-Pd1-P2) and the distance between P1 and P2 in III are greater than those in IV (113.21° vs 102.19°, 3.773 Å vs 3.489 Å). However, this complex III failed to catalyze the enantioselective allenylation under the standard conditions or with AcOH as the protic additive (Fig. 5d ), indicating that the complex III is not really a catalytically active species but provides a stable coordination mode for the palladium catalysis. The X-ray crystal structures of III and IV were then taken as the starting geometries for all the following calculations involving these complexes by restoring the ligand’s amide N-H. Fig. 5: A proposal mechanism and some experiments for Pd-ligand complexes. a A mechanism for the allenylation of pyrazolone. b Synthesis of Pd(II)- DACH-ZYC-Phos-C1 complex III . 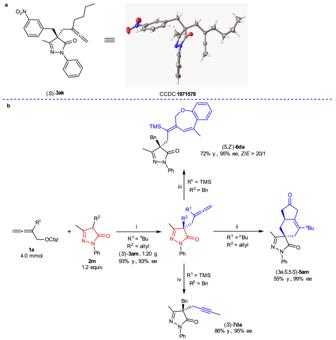Fig. 4: ORTEP representation and sythetic applications. aORTEP representation of (S)-3ak.bThe gram-scale reaction and applications: reaction conditions: (i) Pd2(dba)3•CHCl3(2.5 mol%),DACH-ZYC-Phos-C1(5.0 mol%), toluene, 60 °C, 13 h; (ii) [Rh(CO)2Cl]2(5.0 mol%), AgSbF6(12.5 mol%), CO balloon, toluene, 50 °C, 13 h; (iii) ortho-(propen-2-yl)phenol (3.0 equiv), Pd(OAc)2(7.5 mol%), 2,2’-bipy (7.5 mol%), Cu(OAc)2•H2O (0.5 equiv), toluene, 110 °C, 18 h; (iv) TiCl4(1.5 equiv), dichloromethane, −78 °C, 2.5 h, rt, 5.5 h. TMS trimethylsilyl, Cbz benzyloxycarbonyl, y. isolated yield. c ORTEP representations of Pd(II)-ligand complexes III and IV . 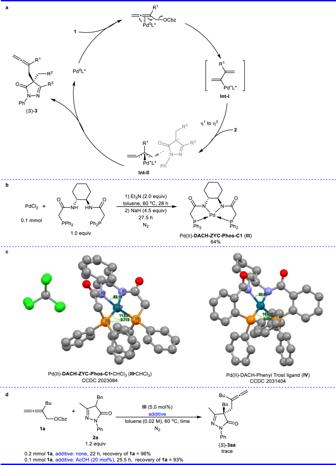Fig. 5: A proposal mechanism and some experiments for Pd-ligand complexes. aA mechanism for the allenylation of pyrazolone.bSynthesis of Pd(II)-DACH-ZYC-Phos-C1complexIII.cORTEP representations of Pd(II)-ligand complexesIIIandIV. H-atoms are omitted for clarity.dThe reaction of pyrazolone2aand allene1awith complexIII. Cbz benzyloxycarbonyl, DACH (1R,2R)-1,2-diaminocyclohexane. H-atoms are omitted for clarity. d The reaction of pyrazolone 2a and allene 1a with complex III . Cbz benzyloxycarbonyl, DACH (1 R ,2 R )-1,2-diaminocyclohexane. Full size image DFT calculations were performed on the enantioselectivity determining C−C bond formation step of the reaction of benzyl buta-2,3-dienyl carbonates 1b with pyrazol-5-one 2a catalyzed by the DACH-ZYC-Phos-C1 -ligated palladium catalyst (see computational methods in the Supplementary Information for details). The reported energies are Gibbs energies that incorporate the effect of the toluene solvent. 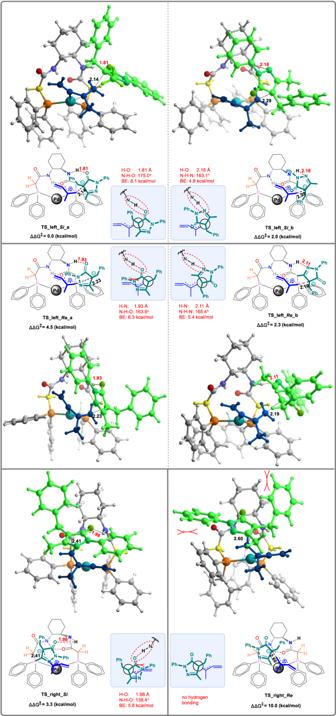Fig. 6: DFT calculations for DACH-ZYC-Phos-C1-ligated palladium catalyst. DFT-optimized structures and relative energies of stereo-determining C−C bond formation transition states of the reaction of1bwith2acatalyzed by theDACH-ZYC-Phos-C1-ligated palladium catalyst. Hydrogen-bonding interactions are shown as red dash lines; selected bond lengths (Å) and bond angles (°) are listed. BE bond energy. 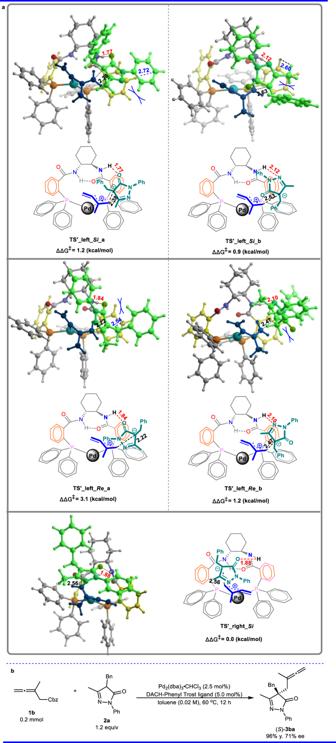Fig. 7: DFT calculations for the DACH-Phenyl-Trost-ligated palladium catalyst. aDFT-optimized structures and relative energies of ee determining C−C bond formation transition states for the reaction of1bwith2acatalyzed by the DACH-Phenyl-Trost-ligated palladium catalyst. Hydrogen-bonding interactions are shown as red dash lines; selected bond lengths (Å) are listed.bThe reaction of1band2awith DACH-Phenyl-Trost ligand. Cbz benzyloxycarbonyl, DACH (1R,2R)-1,2-diaminocyclohexane, y. NMR yield. Figure 6 shows the optimized structures and relative free energies of the competing transition states basing on the endo-methylene- π -allyl palladium complexes [52] (see the Supplementary Information for the other less favorable transition structures with exo-methylene- π -allyl palladium complexes). These transition structures are denoted as TS_left_ Si_ a/b , TS_left_ Re_ a/b , TS_right_ Si , and TS_right_ Re , separately (left/right indicates that the side of methylene moiety referring to the π-allyl Pd unit). Among them, TS_left_ Si _a with the Si -face attack of 2a anion, is found to be the most favorable one, which is consistent with the dominant formation of S -products observed in the experimental studies. Fig. 6: DFT calculations for DACH-ZYC-Phos-C1-ligated palladium catalyst. DFT-optimized structures and relative energies of stereo-determining C−C bond formation transition states of the reaction of 1b with 2a catalyzed by the DACH-ZYC-Phos-C1 -ligated palladium catalyst. Hydrogen-bonding interactions are shown as red dash lines; selected bond lengths (Å) and bond angles (°) are listed. BE bond energy. Full size image The ligand’s right-side amide N-H is available for hydrogen bonding to either the carbonyl oxygen or the hydrazine nitrogen of the approaching 2a anion. The structures of TS_left_ Si _a and TS_left_ Si _b , leading to the formation of the allenylation product with S configuration, are stabilized by the hydrogen bonding forming between the ligand’s N-H with the carbonyl oxygen and the hydrazine nitrogen, separately. In the structure of TS_left_ Si _a , the H···O distance is 1.81 Å, and the bond angle of N − H···O is 175.0°, which are consistent with the common hydrogen bonding parameters [53] . Based on the electron density at the bond critical point, the hydrogen binding energies (BE) were calculated to analyze the strength of the hydrogen bonding [54] . The bond energy of the hydrogen bonding in TS_left_ Si _a was estimated to be about 8.1 kcal/mol. Although the influence of the π/π interactions between the aromatic rings of the ligand and N-Ph pyrazolones on the enantioselectivity could be excluded based on the results of ( S )- 3bu and ( S )- 3bv , we have also tried to analyze the non-covalent interactions (NCI) in TS_left_ Si _a using the Multiwfn [55] , [56] and VMD programs [57] and no obvious π–π interactions are found so far from the analysis (see supplementary information for the NCI plot of TS_left_ Si _a) . The hydrogen bonding in TS_left_ Si _b features a longer H···N distance of 2.18 Å and a smaller N − H···O bond angle of 163.1°, suggesting a weaker interaction, which estimated to be 4.8 kcal/mol. Similarly, hydrogen-bonding interactions also exist in the structure of TS_left_ Re _a and TS_left_ Re _b , which would provide the allenylation product with R configuration. TS_left_ Re _a , is stabilized by the hydrogen bonding formed between the ligand’s N-H and the carbonyl oxygen of 2a anion, which was estimated to be about 6.3 kcal/mol. Moreover, TS_left_ Re _a suffers the unfavorable interaction between 2a anion and the methylene-π-allyl moiety, which have been clearly shown in the Newman projection along the forming C–C bond in Fig. 6 . Both factors contribute to the lower stability of TS_left_ Re _a as compared to TS_left_ Si _a by 4.5 kcal/mol. The bond energy of the hydrogen bonding in TS_left_ Re _b was estimated to be about 5.4 kcal/mol, which is around 2.7 kcal/mol weaker than the one in TS_left_ Si _a (about 8.1 kcal/mol), thus, accounting for the preference of TS_left_ Si _a over TS_left_ Re _b by 2.3 kcal/mol. Furthermore, TS_right_ Si is also stabilized by the hydrogen bonding formed between the ligand’s N-H and the carbonyl oxygen of 2a anion. No corresponding TS is able to be located with hydrogen bonding formed between the ligand’s N-H and the hydrazine nitrogen. The bond energy of the hydrogen bonding in TS_right_ Si was estimated to be about 5.8 kcal/mol. What’s more, the steric repulsions between 2a anion and the methylene- π -allyl moiety destabilize TS_right_ Si . Both factors lead to the less stability of TS_right_ Si than TS_left_ Si_ a by 3.3 kcal/mol. In addition, there is no hydrogen bonding existing in TS_right_ Re . And unfavorable steric interactions between the two phenyl groups of 2a anion and the DACH-ZYC-Phos-C1 ligand further destabilize TS_right_ Re , making it the least stable transition state (10.0 kcal/mol higher in energy than TS_left_ Si_a ). The calculated enantioselectivity, basing on the energy difference between TS_left_ Si_ a and TS_left_ Re_ b of 2.3 kcal/mol, is 94%, which is in perfect agreement with the experimental ee value of 93% (Table 2 , entry 2). Similar calculations were then conducted to compare with DACH-Phenyl-Trost ligand. The optimized structures and relative free energies of the competing transition states of the enantioselectivity-determining C−C bond formation step, associated with the endo-methylene- π -allyl palladium complexes, are illustrated in Fig. 7a , which are denoted as TS’_left_ Si_ a/b , TS’_left_ Re _a/b and TS’_right_ Si , separately. It should be noted that the structure of TS’_right_ Re has not been located successfully, despite all the efforts, probably due to the severe steric repulsions. Different from the DACH-ZYC-Phos-C1 participated reaction, all the transition structures with methylene moiety lying on the left side to the π -allyl Pd unit suffer the steric interactions causing by 2a anion with the phenyl group in phenyl-Trost ligand, which reduce their stability. Nevertheless, via avoiding the unfavorable hindrance caused by the nucleophile 2a anion with the phenyl group in phenyl-Trost ligand, TS’_right_ Si becomes the most favorable transition state. The energy difference between the diastereomeric TS’_right_ Si and TS’_left_ Re_ b is found to be 1.2 kcal/mol. The calculated enantioselectivity of 71% in favor of also the S enantiomer is in agreement with the experimental ee value of 71% (Fig. 7b ). Fig. 7: DFT calculations for the DACH-Phenyl-Trost-ligated palladium catalyst. a DFT-optimized structures and relative energies of ee determining C−C bond formation transition states for the reaction of 1b with 2a catalyzed by the DACH-Phenyl-Trost-ligated palladium catalyst. Hydrogen-bonding interactions are shown as red dash lines; selected bond lengths (Å) are listed. b The reaction of 1b and 2a with DACH-Phenyl-Trost ligand. Cbz benzyloxycarbonyl, DACH (1 R ,2 R )-1,2-diaminocyclohexane, y. NMR yield. Full size image In summary, we have developed a DPPAA-based ligand for the highly chemo- and enantioselective allenylation of pyrazol-5-ones with benzyl 2,3-dienyl carbonates (up to 97% ee). Many synthetically useful functionalities were tolerated under the catalysis of Pd/ DACH-ZYC-Phos-C1 . A rationale has been provided based on the X-ray diffraction studies of Pd(II)- DACH-ZYC-Phos-C1 complex and DFT calculations. In addition, these types of stretchable chiral pockets may also provide flexiblity and show great potential applications in catalytic enantioselective allylation, allenylation, and other reactions. Such studies are being actively pursued in our laboratory with very promising results and will be reported in due courses. General procedure for the catalytic enantioselective allenylation of pyrazol-5-ones To a flame-dried Schlenk flask were added Pd 2 (dba) 3 •CHCl 3 (12.9 mg, 0.0125 mmol), ( R , R )- DACH-ZYC-Phos-C1 (14.3 mg, 0.025 mmol), toluene (5 mL), 1a (131.5 mg, 0.5 mmol)/toluene (11.7 mL), and 2a (158.7 mg, 0.6 mmol)/toluene (8.3 mL) sequentially under nitrogen atmosphere at room temperature. The flask was put into a pre-heated oil bath and the reaction was complete after being stirred at 60 °C for 12 h as monitored by TLC (eluent: petroleum ether/ethyl acetate = 20/1). The resulting mixture was filtrated through a short column of silica gel eluted with ethyl acetate (15 mL × 3). After evaporation, the crude residue was purified by chromatography on silica gel (eluent: petroleum ether (60–90 °C)/ethyl acetate = 60/1) to afford a pure part of ( S )- 3aa and the impure part was further purified by chromatography on silica gel (eluent: petroleum ether (60–90 °C)/ethyl acetate = 40/1). Two-round chromatography afforded ( S )- 3aa (179.5 mg, 96%) as a liquid: 95% ee (HPLC condition: Chiralcel IA column, n -hexane/ i -PrOH = 90/10, 1.0 mL/min, λ = 254 nm, t R (major) = 5.7 min, t R (minor) = 8.9 min); [α] D 20 = −8.2 ( c = 1.25, CHCl 3 ); 1 H NMR (300 MHz, CDCl 3 ) δ 7.55 ( d , J = 8.1 Hz, 2 H, ArH), 7.30 ( t , J = 7.8 Hz, 2 H, ArH), 7.22–7.02 (m, 6 H, ArH), 4.64–4.49 (m, 2 H, = CH 2 ), 3.18 ( d , J = 13.2 Hz, 1 H, one proton of CH 2 ), 2.89 ( d , J = 13.5 Hz, 1 H, one proton of CH 2 ), 2.69 (dt, J 1 = 15.3 Hz, J 2 = 3.3 Hz, 1 H, one proton of CH 2 ), 2.39 ( d , J = 15.0 Hz, 1 H, one proton of CH 2 ), 2.14 (s, 3 H, CH 3 ), 1.93–1.80 (m, 2 H, CH 2 ), 1.43–1.17 (m, 4 H, CH 2 × 2), 0.83 ( t , J = 7.1 Hz, 3 H, CH 3 ); 13 C NMR (75 MHz, CDCl 3 ) δ 205.3, 174.6, 161.4, 137.6, 134.1, 129.1, 128.5, 128.1, 127.2, 124.8, 119.3, 98.3, 77.7, 60.1, 42.8, 36.1, 32.3, 29.4, 22.1, 14.7, 13.8; IR (neat) ν (cm −1 ) 3063, 3031, 2956, 2927, 2859, 1954, 1712, 1597, 1500, 1455, 1440, 1402, 1366, 1123; MS (EI): m/z (%) 372 ([M] + , 31.27), 186 (100); HRMS calcd. for C 25 H 28 N 2 O [M] + : 372.2202; Found: 372.2202.